Max is a repressor of germ cell-related gene expression in mouse embryonic stem cells Embryonic stem cells and primordial germ cells (PGCs) express many pluripotency-associated genes, but embryonic stem cells do not normally undergo conversion into primordial germ cells. Thus, we predicted that there is a mechanism that represses primordial germ cell-related gene expression in embryonic stem cells. Here we identify genes involved in this putative mechanism, by using an embryonic stem cell line with a Vasa reporter in an RNA interference screen of transcription factor genes expressed in embryonic stem cells. We identify five genes that result in the expression of Vasa when silenced. Of these, Max is the most striking. Transcriptome analysis reveals that Max knockdown in embryonic stem cells results in selective, global derepression of germ cell-specific genes. Max interacts with histone H3K9 methyltransferases and associates with the germ cell-specific genes in embryonic stem cells. In addition, Max knockdown results in a decrease in histone H3K9 dimethylation at their promoter regions. We propose that Max is part of protein complex that acts as a repressor of germ cell-related genes in embryonic stem cells. Embryonic stem cell (ESC) lines are pluripotent stem cell lines that are established in culture from early epiblast of preimplantation embryos [1] , [2] , whereas primordial germ cells (PGCs) arise in situ from proximal epiblast of postimplantation embryos as a result of inducing signals from extraembryonic tissues; PGCs migrate into the indifferent embryonic gonads (genital ridges) and eventually become the founder cells that give rise to eggs or sperm. Although both ESCs and PGCs express pluripotency markers (for example, Oct3/4 and Nanog), these cell types differ in important respects. For example, ESCs maintain pluripotency and can give rise to virtually all embryonic cell types; in contrast, PGCs can only give rise to gametes. This difference in developmental potential might result, at least in part, from the expression of germ cell-related genes in PGCs. Indeed, ESCs maintain their identity and do not convert to PGCs when under normal culture conditions; moreover, forced expression of germ cell-specific DAZ (deleted in azoospermia) family proteins in human ESCs resulted in germ cell differentiation and progression in meiosis in culture [3] . Therefore, there may be mechanisms—such as the repression of germ-cell-related gene expression—that separate the cellular status of ESCs from that of PGCs. Here, we performed an RNA interference (RNAi) screen to identify genes involved in the repression of germ-cell-related gene expression in undifferentiated mouse ESCs, and the Max gene was identified as a strong candidate. Max is a well-characterized partner of Myc family proteins, and is known to be required for almost all of the functions of Myc family proteins [4] , [5] . Reportedly, loss of Max in mouse ESCs resulted in loss of the pluripotent state and subsequent apoptosis, and both phenotypes were circumvented by either forced expression of Nanog or cultivation under MAPK/Gsk3 inhibiting (2i) conditions [6] . Max is a member of the E2F6 complex; this complex contains histone methyltransferases and is involved in gene repression via histone H3K9 methylation [7] , [8] , [9] , [10] . We showed that transient knockdown (KD) of the Max gene in ESCs resulted in global and selective expression of germ-cell-related genes; moreover, the Max-mediated repression of these genes in ESCs seemed to be accomplished via histone methylation. RNAi screening To develop a screening system to identify genes that repress germ-cell-related genes in ESCs, we created two ES cell lines that carried either the red fluorescent protein (RFP) or the Venus reporter driven by the promoter from the mouse vasa homologue ( Vasa , also known as Ddx4 ); these lines were designated VR15 and VV3, respectively. Vasa is considered the best marker of differentiated PGCs [11] , [12] . During mouse embryogenesis, PGCs begin to express Vasa just after they colonize the genital ridges, and this expression persists until the onset of meiotic prophase; moreover, Vasa is specifically and exclusively expressed in germ cells throughout development. In addition, Vasa is not expressed in undifferentiated pluripotent cells such as ESCs or cells of the inner cell mass (ICM) or epiblasts; therefore, Vasa reporters are suitable markers of germ-cell differentiation in ESCs. We generated a transgenic (Tg) mouse line using the VR15 (ref. 13 ) ESCs and confirmed that expression of the RFP reporter in the Tg mouse embryos was restricted to PGCs in genital ridges ( Supplementary Fig. S1 ). By utilizing the two ESC lines, each with Vasa reporter, it was possible to use RNAi to screen for genes that, when silenced, resulted in the expression of a Vasa reporter, and such expression may indicate derepression of Vasa ( Fig. 1a ). 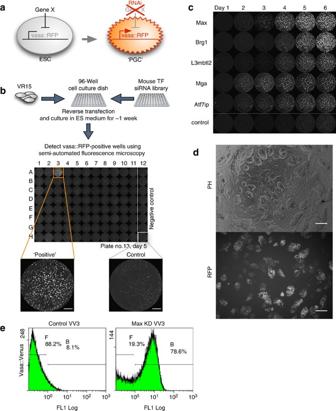Figure 1: An RNAi screen for identifying repressors of germ cell-related gene expression in mouse ESCs. (a) VR15, a mouse ESCs line that carries an RFP reporter driven by theVasapromoter. In this schematic diagram, genes that repress germ-cell-related genes are inactivated by RNAi; consequently, the Vasa::RFP reporter is activated and easily monitored via fluorescence. (b) Top, a schematic diagram of the RNAi screen. The screen was performed using a 96-well format; siRNAs were transfected into VR15 with the reverse method (see Methods). Images of whole-well fluorescent in each well of the 96-well dishes were obtained daily. We tiled the images of 96 wells and searched for the wells that showed significantly brighter fluorescence than negative control wells. Bottom, magnified examples of images of an RFP-positive well and an RFP-negative well. Scale bar, 1 mm. (c) A tiled image that represents the time-dependent changes in RFP fluorescence following KD of each candidate gene in VR15 cells. (d) Phase contrast image (top) and an RFP fluorescence image (bottom) ofMax-KD VR15 cell on day3. Scale bar, 100 μm. (e) Flow cytometry analysis of control VV3 (left) andMax-KD VV3 (right) cells. Robust emergence of a Vasa::Venus-positive cell population was observed in theMax-KD cultures. Figure 1: An RNAi screen for identifying repressors of germ cell-related gene expression in mouse ESCs. ( a ) VR15, a mouse ESCs line that carries an RFP reporter driven by the Vasa promoter. In this schematic diagram, genes that repress germ-cell-related genes are inactivated by RNAi; consequently, the Vasa::RFP reporter is activated and easily monitored via fluorescence. ( b ) Top, a schematic diagram of the RNAi screen. The screen was performed using a 96-well format; siRNAs were transfected into VR15 with the reverse method (see Methods). Images of whole-well fluorescent in each well of the 96-well dishes were obtained daily. We tiled the images of 96 wells and searched for the wells that showed significantly brighter fluorescence than negative control wells. Bottom, magnified examples of images of an RFP-positive well and an RFP-negative well. Scale bar, 1 mm. ( c ) A tiled image that represents the time-dependent changes in RFP fluorescence following KD of each candidate gene in VR15 cells. ( d ) Phase contrast image (top) and an RFP fluorescence image (bottom) of Max -KD VR15 cell on day3. Scale bar, 100 μm. ( e ) Flow cytometry analysis of control VV3 (left) and Max -KD VV3 (right) cells. Robust emergence of a Vasa::Venus-positive cell population was observed in the Max -KD cultures. Full size image We established a screening system to identify genes that, when silenced, resulted in activation of the Vasa gene promoter. VR15 cells were cultured in 96-well plates and subjected to lipofection-mediated transfection with short interfering RNAs (siRNAs). Transfected cells were cultured for 1 week, and RFP fluorescence in each well was recorded daily. We identified wells that had significantly brighter fluorescence than negative control wells ( Fig. 1b ). Whole-well fluorescence images were captured semiautomatically using a microscope equipped with a low-magnification objective lens and a motorized stage. The library used for this screen comprised 864 genes, each of which encoded a transcription factor gene that was expressed in ESCs, as confirmed by transcriptome analysis ( Supplementary Data 1 ). For each of the 864 genes, two independent siRNAs were selected from commercially available, predesigned siRNAs; this library of 1,728 siRNAs was assembled into 96-well format. From the 864 genes, five candidates— Max , Brg1 (also known as Smarca4 ), L3mbtl2 , Mga and Atf7ip —were identified in the screening ( Fig. 1c ). KD of Max , Brg1 , L3mbtl2 or Atf7ip in VR15 cells resulted in a gradual time-dependent increase in RFP fluorescence; in contrast, Mga KD resulted in a relatively acute increase in fluorescence, which was followed by a subtle decline in a later stage ( Supplementary Fig. S2 ). The decline in RFP fluorescence in Mga KD cells was likely due to substantial cell death because many dead cells were seen floating in the wells after 4 days in culture (data not shown). To exclude the possibility that the increases in RFP fluorescence were due to off-target effects of the candidate siRNAs, we confirmed that, for each of the five candidate genes, siRNAs targeting distinct sequences in the messenger RNAs caused the same effects on RFP fluorescence as the original candidate siRNAs ( Supplementary Fig. S3a–e ). In addition, in the case of Max , we simultaneously transfected VR15 cells with siRNA for Max and an expression vector of Max lacking its 3′-UTR that included the target sequences of the siRNAs, and found that the expression vector reversed the siRNA-induced Vasa ::RFP expression ( Supplementary Fig. S3f ). We confirmed that expression of the endogenous Vasa gene was clearly upregulated in Vasa::RFP-positive (VR15) or Vasa::Venus-positive (VV3) cells after KD of each candidate gene 5 days or 3 days after transfection of siRNAs, respectively ( Fig. 2a ), because VR15 cells showed slightly slower induction of the Vasa reporter than VV3 cells (data not shown). 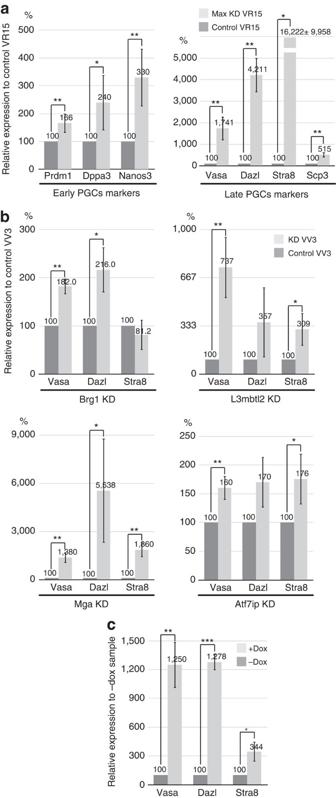Figure 2: KD of candidate genes results in upregulation of germ cell-related genes in ESCs. (a) Expression levels of germ-cell-related genes in FACS-purified Vasa-positiveMax-KD VR15 cells at day 5 were measured using real-time PCR. Relative expression levels are represented; these levels are based on comparisons with control ESCs transfected with the non-silencing control siRNA (AllStars). Early PGC markers (left) and late PGC markers (right) were examined. (b) VV3 cells were subjected to KD of individual candidate genes, and expression of late PGC markers was monitored in FACS-purified cells at day 3. (c) Expression levels of germ-cell-related genes in the ESCs cultured with Doxycyclin (Dox) at day 2 were measured using real-time PCR. In the ESCs,Maxgene was homozygously disrupted, but Max cDNA was introduced inROSA26gene locus together with tetracycline off system6. Relative expression levels are represented; these levels are based on comparisons with control ESCs cultured without Dox. Error bars, s.d. (a,n=4;b,c,n=3) of biological replicates), *P<0.05, **P<0.01, ***P<0.001 (Student’st-test). Figure 2: KD of candidate genes results in upregulation of germ cell-related genes in ESCs. ( a ) Expression levels of germ-cell-related genes in FACS-purified Vasa-positive Max -KD VR15 cells at day 5 were measured using real-time PCR. Relative expression levels are represented; these levels are based on comparisons with control ESCs transfected with the non-silencing control siRNA (AllStars). Early PGC markers (left) and late PGC markers (right) were examined. ( b ) VV3 cells were subjected to KD of individual candidate genes, and expression of late PGC markers was monitored in FACS-purified cells at day 3. ( c ) Expression levels of germ-cell-related genes in the ESCs cultured with Doxycyclin (Dox) at day 2 were measured using real-time PCR. In the ESCs, Max gene was homozygously disrupted, but Max cDNA was introduced in ROSA26 gene locus together with tetracycline off system [6] . Relative expression levels are represented; these levels are based on comparisons with control ESCs cultured without Dox. Error bars, s.d. ( a , n =4; b , c , n =3) of biological replicates), * P <0.05, ** P <0.01, *** P <0.001 (Student’s t -test). Full size image In this study, we focused on Max . Interestingly, ESCs subjected to Max- KD ( Max- KD ESCs) retained an undifferentiated ESC-like appearance ( Fig. 1d ); this finding was surprising given that ESCs lacking all Max reportedly lose the capacity for self-renewal and undergo apoptosis [6] . The reason for this apparent contradiction may be that KD of Max gene expression by siRNA results in incomplete and transient loss of Max protein function ( Fig. 3a ). By day 1 after siRNA transfection, Max protein was decreased to 12% of that at day 0 in VR15 cells, and was subsequently recovered to 37% at day 5 ( Fig. 3a ). Delayed and incomplete recovery of Max protein compared with recovery of Max mRNA suggests post-transcriptional regulation of Max expression ( Fig. 3 ). In the case of VV3 ESCs, Max protein was decreased to 22% at day 3 (data not shown). We confirmed induction of germ-cell-specific genes instead of apoptosis by transient downregulation of Max by using ESCs in which Max gene was homozygously disrupted, but Max cDNA was introduced in ROSA26 gene locus together with tetracycline off system [6] . In this system, we found that presence of 0.1 μg ml −1 of doxycycline for the first one day in culture resulted in transient Max downregulation ( Supplementary Fig. S4 ) and induction of germ-cell-specific genes, but not apoptosis ( Fig. 2c ). Flowcytometric analyses revealed that substantial Vasa ::Venus-positive cell populations emerged in ESC cultures subjected to Max- KD, and the proportion of Vasa ::Venus-positive cells reached 70–80% of all cells in each culture 3 days after transfection of siRNAs ( Fig. 1e ). 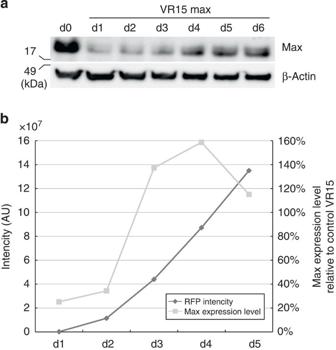Figure 3: Reduction ofMaxexpression in the KD ESCs is transient and incomplete. (a) The time course of changes in Max protein levels inMax-KD VR15. Western blot analyses using antibodies against Max. Max protein was declined to 12% of that at day (d) 0 by d 1, and was subsequently recovered in the KD cells. (b) Changes inMaxmRNA levels inMax-KD VR15 was quantified by real-time PCR and plotted in the graph; the expression level in control VR15 was set as 100%. The time course of changes in RFP intensity ofMax-KD VR15 during culture shown inSupplementary Fig. S2was superimposed on the graph. Principally the same result was obtained in two independent experiments (a,b). Figure 3: Reduction of Max expression in the KD ESCs is transient and incomplete. ( a ) The time course of changes in Max protein levels in Max -KD VR15. Western blot analyses using antibodies against Max. Max protein was declined to 12% of that at day (d) 0 by d 1, and was subsequently recovered in the KD cells. ( b ) Changes in Max mRNA levels in Max -KD VR15 was quantified by real-time PCR and plotted in the graph; the expression level in control VR15 was set as 100%. The time course of changes in RFP intensity of Max -KD VR15 during culture shown in Supplementary Fig. S2 was superimposed on the graph. Principally the same result was obtained in two independent experiments ( a , b ). Full size image Max -KD ESCs show increased PGC marker expression To further investigate the effects of KD of each candidate gene in ESCs, we examined the expression of several representative germ cell markers in ESCs following KD of an individual candidate gene. ESCs were subjected to Max- KD, and the resulting Vasa::RFP-positive cells were isolated using fluorescence-activated cell sorting (FACS) 5 days after transfection of siRNAs; real-time PCR was used to assess the expression of PGC markers in these Vasa::RFP-positive cells. Only modest increases in the expression of three early PGC markers—Prdm1 (refs. 14 ), Dppa3 (refs. 15 , 16 ) and Nanos3 (refs. 17 , 18 )—were observed in the Vasa::RFP-positive cells; however, expression of late-stage PGC markers, including Dazl (refs. 19 , 20 ) and Stra8 (refs. 21 , 22 ), greatly increased. In addition, expression of a meiosis marker, Scp3 (refs. 23 , 24 ), was significantly higher in Vasa::RFP-positive cells than in control cells ( Fig. 2a ). KD of each of the other candidate genes also resulted in increases in the expression of late PGC markers in Vasa ::Venus-positive cells 3 days after transfection ( Fig. 2b ). Next, we evaluated the effects of simultaneous KD of Max and each of the other candidate genes on the expression of the Vasa reporter. Interestingly, simultaneous KD of Max and Brg1 or Atf7ip resulted in enhanced RFP expression relative to KD of Max alone, but simultaneous KD of Max and L3mbtl2 or Mga did not ( Supplementary Fig. S5 ). This observation was consistent with the idea that Max, Mga and L3mbtl2 function together in the same complex to repress expression of germ-cell-related genes; this hypothesis is discussed in more detail below [7] . Upregulated meiosis and spermatogenesis genes in Max- KD ESCs To assess the expression profile of ESCs following Max- KD more comprehensively, we used FACS to purify Vasa::Venus-positive ESCs following Max- KD, and used microarray analysis to compare the transcriptome of these Vasa::Venus-positive cells with that of control ESCs. There were 447 and 313 genes for which expression was at least 2-fold higher or lower in the Vasa ::Venus-positive ESCs than in control ESCs, respectively ( t -test P <0.01, n =3) ( Fig. 4a , Supplementary Tables S1 and S2 ). The set of 447 upregulated genes included all four late-stage PGC-specific genes that were assessed in the real-time PCR analysis ( Fig. 2 ). Gene ontology (GO) analysis of these genes revealed that germ-cell-related GO terms (for example, meiosis, spermatogenesis, germ plasm) were significantly enriched among the GO terms associated with these 447 genes ( Supplementary Table S3 ), while germ-cell-related GO terms were not enriched among the downregulated genes ( Supplementary Table S4 ). Of the 447 upregulated genes, 62 exhibited more than a 10-fold increase in expression in the Vasa::Venus-positive cells; in mice, knockout (KO) of any 1 of 12 of these 62 genes results in a meiosis-related or spermatogenesis-related phenotype (Mouse Genome Informatics http://www.informatics.jax.org/ ). Of the remaining 50 genes, 6 were expected to have a function in spermatogenesis or meiosis based on expression pattern or molecular characteristics (Mouse Genome Informatics; Fig. 4b , Supplementary Table S1 ). Therefore, it seemed that germ-cell-related genes, especially spermatogenesis- and meiosis-related genes, were globally derepressed in the Vasa::Venus-positive cells. In contrast, expression of pluripotency markers (for example, Oct3/4 (also known as Pou5f1) and Nanog) was not affected by Max- KD ( Supplementary Fig. S6 ). 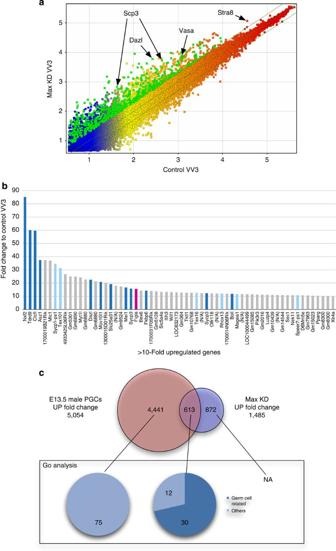Figure 4: Microarray analysis reveals that genes involved in meiosis and spermatogenesis are upregulated inMax-KD ESCs. (a) Scatter plot of control VV3 (xaxis) andMax-KD VV3 (yaxis). Green dots indicate genes that were upregulated in bothMax-KD VV3 and E13.5 PGCs; expression in control ESCs was used as the baseline. The late PGC markers analysed in Fig. 2 are indicated by arrows. Green lines indicate 2-fold upregulation and downregulation. (b) Fold changes in the expression of the top 62 genes, each of which showed more than 10-fold upregulation inMax-KD VV3 compared with control VV3. Blue bars, genes for which gene knockout in mice resulted in meiosis-specific defects, spermatogenesis-specific defects, or both. Light blue bars, genes expected to be involved in meiosis, spermatogenesis, or both. Pink bar, a gene for which gene KO in mice resulted in oogenesis-specific defects. (c) Top, a Venn diagram of the number of genes upregulated in PGCs andMax-KD ESCs. Bottom, result of GO analysis of genes in the intersection or complementary sets from the Venn diagram. Numbers of significantly enriched GO terms are presented in pie graph. Only genes in the intersection showed significant enrichment for germ-cell-related GO terms. NA, not applicable. Figure 4: Microarray analysis reveals that genes involved in meiosis and spermatogenesis are upregulated in Max -KD ESCs. ( a ) Scatter plot of control VV3 ( x axis) and Max -KD VV3 ( y axis). Green dots indicate genes that were upregulated in both Max -KD VV3 and E13.5 PGCs; expression in control ESCs was used as the baseline. The late PGC markers analysed in Fig. 2 are indicated by arrows. Green lines indicate 2-fold upregulation and downregulation. ( b ) Fold changes in the expression of the top 62 genes, each of which showed more than 10-fold upregulation in Max -KD VV3 compared with control VV3. Blue bars, genes for which gene knockout in mice resulted in meiosis-specific defects, spermatogenesis-specific defects, or both. Light blue bars, genes expected to be involved in meiosis, spermatogenesis, or both. Pink bar, a gene for which gene KO in mice resulted in oogenesis-specific defects. ( c ) Top, a Venn diagram of the number of genes upregulated in PGCs and Max -KD ESCs. Bottom, result of GO analysis of genes in the intersection or complementary sets from the Venn diagram. Numbers of significantly enriched GO terms are presented in pie graph. Only genes in the intersection showed significant enrichment for germ-cell-related GO terms. NA, not applicable. Full size image To better understand the relationship between PGCs and ESCs lacking Max, we compared the transcriptomes of PGCs from E13.5 mouse embryos and of Max -KD ESCs with that of control ESCs. Using transcriptome of control ESCs as a reference, genes upregulated in the PGCs or in Max- KD ESCs were identified (5,054 and 1,485 genes, respectively; >2-fold change, one-way analysis of variance P <0.01). Three distinct subsets of these upregulated genes were subjected to GO analysis; these subsets were the 613 genes that were upregulated in both PGCs and Max- KD ESCs, the 4,441 genes that were upregulated in only PGCs, and the 872 genes that were upregulated in only Max- KD ESCs ( Fig. 4c ). Intriguingly, germ-cell-related GO terms were preferentially enriched among the terms associated with genes upregulated in both PGCs and Max -KD ESCs, and no GO terms related to specialized biological processes were found among the terms associated with genes upregulated only in PGCs ( Fig. 4c , Supplementary Tables S5 and S6 ). Moreover, no GO terms were enriched among the terms associated with genes upregulated only in Max -KD ESCs. Therefore, it can be said that germ-cell-specific genes were upregulated both in Max -KD ESCs and PGCs; however, genes that are not related to germ cells may have been aberrantly upregulated in Max -KD ESCs, or Max -KD ESCs may exhibit upregulation of genes required in the later stages of germ cell differentiation. In addition, genes that do not have germ-cell-specific functions but are required for maintenance of germ cells may be upregulated specifically in PGCs. Max interacts with histone H3K9 methyltransferases During embryogenesis, chromosomes in developing PGCs undergo a variety of epigenetic modifications [25] , including a global reduction of histone H3 lysine 9 di- and tri-methylation (H3K9me2, H3K9me3) [26] , [27] , which are regarded as repressive histone modifications. We used antibodies that specifically recognize histone H3K9me2 and H3K9me3 to assess whether H3K9 methylation was lower in Max- KD ESCs than in control cells. On the basis of the western blotting analysis, we found that methylation levels of histone H3K9 was decreased in Max -KD VR15 ESCs by day 3 after transfection of siRNA though the amount of total histone H3 was not changed ( Fig. 5a ). Additionally, immunostaining of Max -KD ESCs with anti-histone H3K9me2 antibodies revealed that expression of H3K9me2 was lower in Vasa::Venus-positive cells than in control cells ( Fig. 5b , arrowheads). Therefore, Max -KD seemed to cause a global reduction of histone H3K9 methylation level in ESCs. 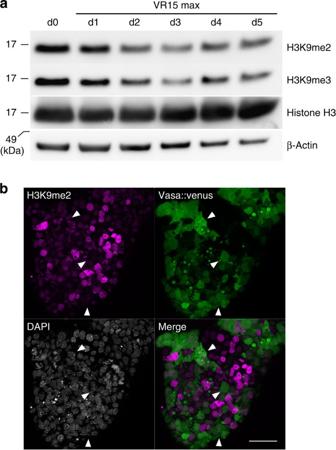Figure 5: Demethylation of histone H3K9 inMax-KD ESCs. (a) Western blot analyses ofMax-KD VR15 using antibodies against histone H3K9me2 and H3K9me3. Substantial reduction of methylated histone H3K9 levels inMax-KD VR15 was observed by day 3 after transfection of siRNA. Principally the same result was obtained in two independent experiments. (b) Immunofluorescence analysis ofMax-KD VV3 using anti-histone H3K9me2 antibody. Most of Vasa::Venus-positive cells were H3K9me2 negative (arrowheads); only 2.2% of the Vasa::Venus-positive cells were H3K9me2 positive, whereas 31.4% of Vasa::Venus-negative cells were H3K9mes positive. Scale bar, 50 μm. Figure 5: Demethylation of histone H3K9 in Max -KD ESCs. ( a ) Western blot analyses of Max -KD VR15 using antibodies against histone H3K9me2 and H3K9me3. Substantial reduction of methylated histone H3K9 levels in Max -KD VR15 was observed by day 3 after transfection of siRNA. Principally the same result was obtained in two independent experiments. ( b ) Immunofluorescence analysis of Max -KD VV3 using anti-histone H3K9me2 antibody. Most of Vasa::Venus-positive cells were H3K9me2 negative (arrowheads); only 2.2% of the Vasa::Venus-positive cells were H3K9me2 positive, whereas 31.4% of Vasa::Venus-negative cells were H3K9mes positive. Scale bar, 50 μm. Full size image Interestingly, three of the five candidate gene products, Max, L3mbtl2 and Mga, are the components of E2F6 complex [7] , [8] , [9] , [10] , which also contains two histone H3K9-specific methyltransferases (Ehmts), G9a and GLP. The complex functions in gene silencing in G0 phase of cell cycle via Ehmt-mediated methylation of histone H3K9. We postulated that Max acted with Ehmts to methylate histone H3K9 and consequently repress germ-cell-related genes in ESCs; we explored this possibility via biochemical analyses. First, we examined interactions between Max and Ehmts in mouse ESCs via co-immunoprecipitation assays by using an anti-Max antibody. We immunoprecipitated Max protein from undifferentiated mouse ESCs and found that both the GLP and the G9a protein were co-immunoprecipitated with Max ( Fig. 6a , Supplementary Fig. S7 ), while reduction of Max protein resulted undetectable GLP or G9a in the precipitates ( Fig. 6a , Supplementary Fig. S7 ). By contrast, interaction between Max and Ezh2, a histone H3K27-specific methyltransferase, was not detected ( Fig. 6b , Supplementary Fig. S7 ), indicating that interaction between Max and G9a/GLP is specific. 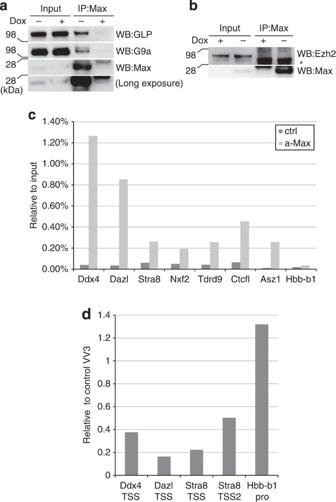Figure 6: Max protein associates with histone H3K9 methyltransferases and the promoter regions of PGC-related genes. (a,b) Immunoprecipitated samples using anti-Max antibody were analysed on western blots. We used theMax-KO ESCs with Max cDNA introduced inROSA26gene locus together with tetracycline off system6. TheMax-null ESCs did not express the Max protein in the presence of 1 μg ml−1doxycycline (Dox). GLP and G9a were immunoprecipitated with anti-Max antibody only in the absence of Dox (a), but Ezh2 was not (b). Max protein was only present when Dox was absent; therefore, these observations strongly supported the conclusion that Max specifically interacted with GLP and G9a in ESCs. Principally the same result was obtained in two independent experiments (a,b). Asterisk inbindicates a non-specific band. (c) ChIP assays involving anti-Max antibodies and undifferentiated VV3 were used to examine the association of Max protein with promoter region of germ-cell-related genes. Relative ratios of the immunoprecipitated chromatin to input chromatin were determined by real-time PCR. The data shown are representative of data from three independent experiments. (d) ChIP assays involving anti-histone H3K9me2 antibody andMax-KD VV3 were used to examine the amount of methylated histone H3K9 in the promoter region of late PGC marker genes, and ofhaemoglobin β(Hbb-b1) gene as a negative control. There was a significant reduction in methylated histone H3K9 in germ-cell-related genes inMax-KD VV3 cells compared with control VV3 cells. By contrast, no reduction was observed inHbb-b1. The amount of methylated histone H3K9 relative to input were calculated and ratios of the amount in Max-KD VV3 to control VV3 were represented. Shown is a representative of two independent experiments. IP, immunoprecipitation; US, upstream region; WB, western blot. Figure 6: Max protein associates with histone H3K9 methyltransferases and the promoter regions of PGC-related genes. ( a , b ) Immunoprecipitated samples using anti-Max antibody were analysed on western blots. We used the Max -KO ESCs with Max cDNA introduced in ROSA26 gene locus together with tetracycline off system [6] . The Max -null ESCs did not express the Max protein in the presence of 1 μg ml −1 doxycycline (Dox). GLP and G9a were immunoprecipitated with anti-Max antibody only in the absence of Dox ( a ), but Ezh2 was not ( b ). Max protein was only present when Dox was absent; therefore, these observations strongly supported the conclusion that Max specifically interacted with GLP and G9a in ESCs. Principally the same result was obtained in two independent experiments ( a , b ). Asterisk in b indicates a non-specific band. ( c ) ChIP assays involving anti-Max antibodies and undifferentiated VV3 were used to examine the association of Max protein with promoter region of germ-cell-related genes. Relative ratios of the immunoprecipitated chromatin to input chromatin were determined by real-time PCR. The data shown are representative of data from three independent experiments. ( d ) ChIP assays involving anti-histone H3K9me2 antibody and Max -KD VV3 were used to examine the amount of methylated histone H3K9 in the promoter region of late PGC marker genes, and of haemoglobin β ( Hbb-b1 ) gene as a negative control. There was a significant reduction in methylated histone H3K9 in germ-cell-related genes in Max -KD VV3 cells compared with control VV3 cells. By contrast, no reduction was observed in Hbb-b1 . The amount of methylated histone H3K9 relative to input were calculated and ratios of the amount in Max-KD VV3 to control VV3 were represented. Shown is a representative of two independent experiments. IP, immunoprecipitation; US, upstream region; WB, western blot. Full size image To confirm the requirement of GLP and G9a for repression of germ-cell-specific genes, we examined the expression of Vasa , Dazl and Stra8 in G9a or GLP-KO ESCs [28] , [29] , [30] , and found that their expression was significantly upregulated in the KO ESC as in Max-KD ESC ( Fig. 7a ). Previous studies demonstrated that KO phenotypes were reversed in the G9a or GLP-KO ESCs with forced expression of G9a or GLP, respectively [28] , [29] , [30] , and we confirmed that the expression of Vasa , Dazl and Stra8 was reversed in those rescued ESCs ( Fig. 7a ). 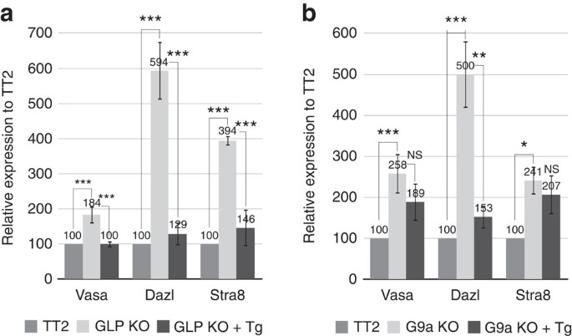Figure 7: Knockout of GLP and G9a results in upregulation of germ-cell-related genes in ESCs. Expression levels of germ-cell-related genes in (a) GLP- or (b) G9a -knockout ESCs, and in those cells rescued by the expression vectors of GLP and of G9a, respectively, were measured using real-time PCR. Relative expression levels are represented; these levels are based on comparisons with parent TT2 ESCs. Error bars, s.d. (a,b,n=3) of biological replicates), *P<0.05, **P<0.01, ***P<0.001, NS, not significant (Student’st-test). Figure 7: Knockout of GLP and G9a results in upregulation of germ-cell-related genes in ESCs. Expression levels of germ-cell-related genes in ( a ) GLP- or ( b ) G9a -knockout ESCs, and in those cells rescued by the expression vectors of GLP and of G9a, respectively, were measured using real-time PCR. Relative expression levels are represented; these levels are based on comparisons with parent TT2 ESCs. Error bars, s.d. ( a , b , n =3) of biological replicates), * P <0.05, ** P <0.01, *** P <0.001, NS, not significant (Student’s t -test). Full size image Next, to assess the possibility that Max directly regulated expression of germ-cell-related genes, we examined the association between the Max protein and the transcription start sites (TSSs) of putative target genes via chromatin immunoprecipitation (ChIP) assays involving anti-Max antibodies. We found that the Max protein was enriched at the TSSs of many germ-cell-related genes—including Vasa , Dazl , Stra8 , Scp3 , and the four genes that were most upregulated in the Max -KD ESCs ( Fig. 6c ), while enrichment of Max protein was not observed at the TSS of haemoglobin-β gene ( Hbb-b1 ) whose expression in ESCs was very low and was not changed by Max -KD ( Supplementary Fig. 6 ). We hypothesized that Max repressed the expression of these genes facilitating repressive histone modifications, especially H3K9 methylation. We tested this hypothesis by assessing the methylation status of three germ-cell-related genes in Max -KD ESCs in a ChIP assay involving anti-histone H3K9me2 antibodies. This ChIP assay revealed that the levels of histone H3K9 dimethylation in the TSS of Vasa, Dazl , Stra8 and Scp3 were markedly lower in Max -KD ESCs than in control cells, while it was not significantly affected in the TSS of Hbb-b1 ( Fig. 6d ). On the basis of these findings, we propose that Max forms complex with Ehmts and probably with L3mbtl2, Mga as well in undifferentiated ESCs, and represses the expression of germ-cell-related genes via repressive histone modification, namely H3K9 methylation. We also examined the expression of Max in purified PGCs specifically expressing mil1-GFP transgene [31] and GFP-negative surrounding somatic cells in embryos and in ES cells. We found that Max was expressed in PGCs, and its expression level was significantly higher than that in ES cells and in the somatic cells ( Fig. 8a ). A previous study [27] demonstrated that the expression of G9a and GLP was undetectable in PGCs at E9.5, and we confirmed that G9a expression was undetectable in mil1-GFP -positive PGCs at E10.5 ( Fig. 8b ). As representative germ-cell-related genes such as Vasa , Dazl and Stra8 are expressed in PGCs between E11.5 and E14.5 ( [11] , [32] , [33] ), the results suggest that Max is not functional with regard to the repression of germ cell gene because of the lack of its partner molecules, GLP and G9a in PGCs. 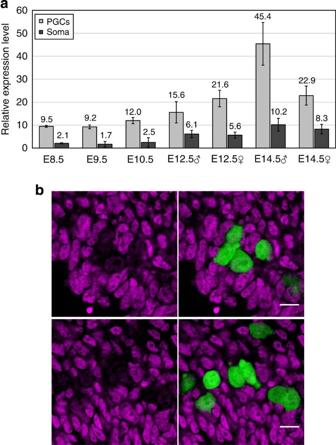Figure 8: The expression ofMaxand G9a in PGCs. (a) Relative expression levels ofMaxin purified GFP-positive PGCs and in the adjacent GFP-negative somatic cells frommil1-GFPTg embryos at different embryonic stages compared with its expression in E14-1 ES cells, which was set as 1.0. Error bars, s.d. (n=3) of biological replicates. (b) Immunostaining of E10.5 PGCs for G9a (magenta). PGCs were detected by the expression ofmil1-GFPtransgene (green), shown in the merged images in the right panels. G9a expression was undetectable or very low in GFP-expressing PGCs. Scale bar, 10 μm. Figure 8: The expression of Max and G9a in PGCs. ( a ) Relative expression levels of Max in purified GFP-positive PGCs and in the adjacent GFP-negative somatic cells from mil1-GFP Tg embryos at different embryonic stages compared with its expression in E14-1 ES cells, which was set as 1.0. Error bars, s.d. ( n =3) of biological replicates. ( b ) Immunostaining of E10.5 PGCs for G9a (magenta). PGCs were detected by the expression of mil1-GFP transgene (green), shown in the merged images in the right panels. G9a expression was undetectable or very low in GFP-expressing PGCs. Scale bar, 10 μm. Full size image We recovered three members of the E2F6 complex—Max, L3mbtl2 and Mga [7] —in a screen for genes that repress germ-cell-related genes in ESCs ( Fig. 1 ). A number of studies demonstrated that E2F6 complex in different kinds of cells often contained Max, Mga, L3mbtl2, GLP and G9a (refs. 7 , 8 , 8 , 10 ). Interestingly, several reports show that E2F6 acted as a repressor of germ-cell-related genes in somatic tissues [34] , [35] , [36] , [37] . However, our analysis showed that inhibition of E2F6 in mouse ESCs did not result in derepression of the Vasa promoter and that Max, Mga and L3mbtl2 were the only members of the E2F6 complex whose inhibition resulted in activation of Vasa promoter ( Supplementary Data 1 ). Therefore, a complex that is similar to but distinct from the E2F6 complex may act as a repressor of germ-cell-related genes in ESCs. As Max is also expressed in embryonic ( Fig. 8a ) and adult somatic cells [38] , Max-containing protein complexes are likely involved in repression of germ-cell-related genes in somatic cells as well. Additionally, mutations in Drosophila homologue of L3mbtl2 resulted in ectopic expression of germ-cell-related genes in larval brain [39] . Therefore, the role of L3mbtl2 in the repression of germ-cell-related gene seems to be conserved between species. Intriguingly, the human ortholog of Atf7ip , another candidate gene, facilitates di- to tri-methylation of histone H3K9 by the SETDB1 (SET domain, bifurcated 1) methyltransferase [40] . As KD of Atf7ip enhanced derepression by Max -KD in ESCs ( Supplementary Fig. S5 ), Atf7ip may act independently from Max, L3mbtl and Mga. Our siRNA screen included Myc family genes, that is, N-myc, L-myc, B-myc, Max, Mlx, Mxd3, Mxi and Mga ( Supplementary Data 1 ), and we additionally tested siRNA for c -myc, s-myc, Mxd1, Mxd4 and Mnt , but only Max- and Mga-KD resulted the Vasa reporter induction. Max often interact with Myc, Mxds or Mnt proteins and associate with E-box sequences to control transcription, but E-box sequences were not found in the vicinity of Stra8 and Ctcfl, in which Max was associated ( Fig. 6c ). Therefore, it is likely that Max functions as a germ cell gene repressor via interacting with G9a/GLP rather than with Myc, Mxd or Mnt. Although binding sequence specificity of the Max/G9a/GLP complex is currently unknown, this complex may preferentially associate with specific sequences present within the promoter regions of germ-cell-specific genes. The ESCs subjected to Brg1 -KD differed from those subjected to KD of any of the other four candidate genes in two respects: the Brg1 -KD ESCs had a partially differentiated colony morphology (data not shown), and upregulation of the Vasa reporters was relatively delayed following KD of Brg1 ( Supplementary Fig. S2 ). Brg1 is an ATP-dependent chromatin remodelling factor and a core component of the BAF (Brg1/Brahma-associated factors) complex. ESCs have a special type of BAF complex, called esBAF [41] , [42] , [43] , that has a critical role in the maintenance of pluripotency. Some genes encoding proteins in the esBAF complex were included in the library used in our initial screen; nevertheless, Brg1 was the only one of these esBAF complex genes that was recovered in our screen for genes involved in germ-cell-related gene derepression ( Supplementary Data 1 ). Therefore, Brg1 may have a role in the repression of germ-cell-related genes that is independent from its esBAF-mediated role in ESCs; accordingly, Brg1 -KD ESCs exhibited both differentiated colony morphology and germ-cell-related gene derepression. When Max is completely eliminated from ESCs, the cells lose pluripotency and undergo apoptosis [6] . However, we showed that transient KD of Max in ESCs resulted in derepression of germ-cell-related gene rather than differentiation and apoptosis ( Fig. 1d , 3 ). This discrepancy may indicate that Max acts in a dose-dependent manner. Interestingly, Oct3/4 regulates the fate of ESCs in a dose-dependent manner [44] . If Oct3/4 expression is increased more than 1.5-fold above baseline expression levels in ESCs, these cells differentiate into primitive endodermal or mesodermal cells, and a reduction of Oct3/4 expression to <50% of baseline expression levels results in dedifferentiation into trophectoderm. The expression level of Max may affect the fate of ESCs in a similar way. Reduction of Max protein to about 10–40% of baseline expression levels ( Fig. 3a ) resulted in activation of germ-cell-related genes, and complete repression results in loss of pluripotency and apoptosis. Reportedly, Max expression is ubiquitous in mouse embryos throughout early development and in the pre- and peri-implantation stages [45] . Given this Max expression pattern, our observations indicated that one in vivo function of Max in early development might be repression of germ-cell-related genes in the ICM, which consists of pluripotent cells. Interestingly, PGC-specific genes are transiently induced as ICM cells become ESCs in culture [1] , [46] . As the ICM and ESC lines have distinct cellular characteristics, it is likely that Max prevents cells of the ICM from adopting a ESC-like cellular status in embryos. Alternatively, Max might suppress precocious development of germ cells in peri-implantation embryos. PGCs also express Max at even higher levels than that in ES cells in spite of the expression of germ-cell-related genes. However, PGCs lack GLP and G9a, critical partner molecules of Max, which may ensure the expression of germ-cell-related genes in PGCs. Taken together, our results indicate that Max and its associated molecules have a pivotal role on repression of germ-cell-related genes in pluripotential stem cells. Our study demonstrated that Max -KD ESCs exhibited selective derepression of genes related to meiosis and spermatogenesis. Thus, Max -KD ESCs may have transformed into a germ-cell-like state. To test this possibility, we first examined whether Max -KD ESCs proceeded to meiosis, but they showed no sign of haploid cells by flow cytometry ( Supplementary Fig. 8a ) and of formation of synaptonemal complex by localization of Scp3 protein though increased Scp3 showed dot-like localization in nucleus of Max -KD ESCs, resembling that in pre-meiotic PGCs [47] ( Supplementary Fig. 8b ). In addition, we transplanted FACS-purified Vasa -positive Max -KD ESCs into testes of mutant newborn mice (azoospermia W/W v ) [48] . Very few teratomas formed (3 out of 28 or 1 out of 8 recipient testes transplanted Max -KD VR15 or VV3 developed teratmas, respectively), but the transplanted cells rarely contributed to spermatogenesis, though transplanted PGCs showed spermtogeneisis ( Supplementary Fig. S9 ). Therefore, although Max -KD seemed to eliminate the pluripotency of ESCs, it did not elicit a true germ-cell-like state in these cells at least in the experimental conditions in this study. In addition, we cannot exclude a possibility that transplanted cells may have been unable to colonize seminiferous tubules because these cells were rarely observed in recipient testes of adults. To explain these observations, we hypothesize that Max may only regulate those genes that have specialized functions in germ cells, but not the genes that are required for, but not specific to, germ cells ( Fig. 4c ). Max -KD ESCs may partially convert to PGCs, and additional changes in gene expression (for example, changes related to germ cell metabolism) may be required for complete conversion to PGCs. Alternatively, this incomplete conversion might be attributed to the epigenetic status of genomic DNA in Max -KD ESCs. PGCs undergo erasure of genome imprinting during development in vivo [25] , [26] . We surveyed the status of genome imprinting in Max -KD ESCs, and found that no erasure of imprinting was observed in the H19 or Igf2r region ( Supplementary Fig. S10 ). Max -KD ESCs might be in a transition state between ESCs and PGCs, and additional modifications (for example, more extensive erasure of genomic imprinting) might result in a complete conversion of Max -KD ESCs to PGCs. In recent years, derivation of germ cells from ESCs has been investigated extensively [3] , [49] , [50] , [51] , [52] , [53] ; however, autonomous differentiation or guided differentiation were utilized in these reports. Notably, ESCs and PGCs express many of the same pluripotency markers. Therefore, we consider that direct conversion may be the best way to derive germ cells from ESCs. Our finding indicated that it may be possible to convert ESCs into germ cells directly, and that the transient KD of the Max gene might be an important step in the direct conversion of ESCs into germ cells. ESCs culture VR15 ESCs were cultured in KO DMEM (Gibco 10829-018) supplemented with 15% fetal bovine serum (FBS), 4 mM L -glutamine, 0.01 mM non-essential amino acids, 0.1 mM β-mercaptoethanol, 1,000 U ml −1 LIF (ESGRO Millipore ESG1107) on mouse embryonic fibroblasts inactivated with mitomycin C. VV3 ESCs were cultured in Glasgow MEM supplemented with 15% KnockOut Serum Replacement (Gibco 10828-028), 1% FBS, 2 mM L -Glutamine, 0.1 mM non-essential amino acids, 1 mM sodium pyruvate, 0.11 mM β-mercaptoethanol and 1,000 U ml −1 LIF on inactivated STO feeder cells. Max-, GLP- and G9a-null ESCs were cultured as described previously [6] , [28] . All ESC lines were maintained at 37 °C in 5% CO 2 . RNAi siRNAs were transfected into cells using Lipofectamine RNAiMAX (Invitrogen 13778) and the reverse method according to the manufacturer’s instructions. Briefly, transfection in 96-well format was carried out as follows. Lipofectamine RNAiMAX (0.5 μl) and siRNA (12 pmol) were diluted with 20 μl OptiMEM and incubated for 20 min. An aliquot of 7,500 ESCs in 100 μl of ES medium was added to each Lipofectamine/siRNA mixture and mixed briefly. The ESCs/siRNA mixtures were seeded onto 96-well plates pre-seeded with feeder cells. The cells were incubated for 24 h and fed with normal ES medium. siRNAs were designed and manufactured by Qiagen. IDs of siRNAs used in this report are listed in Supplemetary Methods . RNAi screen A list of mouse genes encoding transcription factor were obtained from the Riken Transcription Factor Database: TFdb [54] ( http://genome.gsc.riken.jp/TFdb/ ). From the list, genes that were confirmed to be expressed in ESCs were selected based on transcriptome analysis of E14-1 available from HiCEP (high-coverage gene expression profiling) database [55] ( http://hicepweb.nirs.go.jp/peakdb/query?request=dbmain ). The list was revised by manually; ultimately, 864 genes were selected. Two independent predesigned siRNAs for each gene were selected and purchased from Qiagen. The list of genes that constitute the siRNA library used in the screen is presented in Supplementary Data 1 . VR15 ESCs were transfected with individual siRNAs in a 96-well format as described above; transfected cells were cultured for 1 week. Whole-well RFP fluorescent images were obtained semiautomatically using the Leica AS MDW system equipped with a motorized stage, a CO 2 incubator, a X2.5 objective lens, a cooling CCD camera (Photometrics CoolSNAP HQ) and zoom C-mount adaptor (Leica 11 541 517) used at ~X0.35 magnification. The images were flattened, enhanced and tiled using the ImagePro Plus software (Roper Scientific). Wells with significantly brighter fluorescence than negative control wells were review by direct visual inspection. Collection of PGCs from embryos All the animal experiments were performed under the ethical guidelines of the Tohoku University, and animal protocols were reviewed and approved by the Tohoku University Animal Studies Committee. MCH were purchased from Japan SLC, Inc. Oct4ΔPE-GFP [56] and mil1-GFP [31] Tg mice were maintained in a C57BL/6J genetic background. These mice were kept and bred in the animal unit of the Institute of Development, Aging and Cancer (Tohoku University); this facility is environmentally controlled and specific pathogen free. To obtain embryos, female MCH mice were mated with Oct4ΔPE-GFP or mil1-GFP Tg males; dams were killed at appropriate embryonic days (noon on the day of plug release is embryonic day 0.5 [E0.5]). The genital ridges were dissected from the embryo and incubated in trypsin–EDTA solution for 30 min at 37 °C. The cells in tissue samples were dissociated by pipetting and filtered through a 40-μm pore-size cell strainer (BD Falcon). For real-time PCR of PGCs, GFP-positive PGCs were manually isolated form mil1-GFP Tg embryos under a fluorescent microscope. Fluorescence-activated cell sorting Cells expressing fluorescent protein were collected from suspensions of ESCs or PGCs using an EPICS ALTRA unit (Beckman Coulter). Vasa::RFP-positive cells from Max -KD VR15 were collected on day 5. Vasa::Venus-positive cells from Max-, Mga -, L3mbtl2 - or Atf7ip -KD VV3 were collected on day 3, and Vasa::Venus-positive cells from Brg1 -KD VV3 were collected on day 5. For DNA content analysis, single cell suspensions of ESCs were fixed with ice-cold 70% ethanol, treated with RNase and stained with propidium iodide. DNA content of the stained cells were analysed by FC500 (Beckman Coulter). RNA preparation and real-time PCR Total RNA sample were purified using the Qiagen RNeasy Plus mini kit or the RNeasy micro kit according to the manufacturers’ instruction. RNAs were reverse-transcribed using SuperScript III and random primers. Expression levels of PGC marker genes were quantified using the TaqMan Gene Expression Assay (Applied Biosystems). Expression levels of each gene were normalized to Gapdh expression using standard curve method or comparative CT method. Probes used in this paper were: Max Mm00484800_m1; Nanos3 Mm00808138_m1; Prdm1 Mm00476128_m1; Dppa3 Mm00836373_g1; Ddx4 Mm00802445_m1; Dazl Mm00515630_m1; Stra8 Mm00486473_m1; Sycp3 Mm00488519_m1; Gapdh 4352932E. Microarray analysis Total RNA (100 ng) from each sample was analysed. Samples were prepared using the Agilent Low Input Quick Amp Labeling Kit (one colour) (5190-2305); probes were hybridized onto the Agilent Whole Mouse Genome Oligo DNA microarray kit Ver 2.0 (Agilent G4846A) according to the manufacturer’s instructions. The microarrays were scanned using the Agilent DNA microarray scanner (Agilent G2505C); the spot signals were quantified using Feature Extraction software. The datasets were analysed by GeneSpringGX (Agilent). Each cell type was analysed in three biological replicate. Multiple testing correction has been performed using the Benjamini-Hochberg false-discovery rate correction. Western blot Protein extracts were subjected to electrophoresis on NuPAGE 10% Bis-Tris Gels (Invitrogen NP0302), and transferred to polyvinylidene difluoride membrane (Millipore Immobilon-P). Membranes were incubated with the indicated antibodies in 5% skim milk/PBS for overnight at 4 °C. After washing, the membranes were incubated with horseradish peroxidase-labelled secondary antibodies. The membranes were washed again and the signals were detected using the ECL system (GE Healthcare). Immunofluorescence For staining of histone H3K9me2, ESCs grown on CellDesk LF (Sumitomo Bakelite) pre-seeded with feeder cells were fixed with 4% paraformaldehyde in PBS for 1 h, permeabilized with 0.5% Triton-X in PBS for 5 min, and then incubated with blocking solution (10% FBS, 1% BSA, 0.1% Triton-X in PBS) for 1 h at room temperature. The cells were incubated with primary antibody in the blocking solution overnight at 4 °C. The cells were washed, then incubated with secondary antibody for 1 h at room temperature. Cells were washed again and mounted with VECTASHIELD (Vector Laboratories). The specimens were observed under a confocal laser scan microscopy (Leica TCS SP2). To stain G9a in mouse embryos, E10.5 mil1-GFP Tg embryos were dissected at middle of the body and the posterior half fragments were fixed with 4% paraformaldehyde in PBS at 4 °C overnight, then incubated sequentially in 20% sucrose, 1:1 mixture of 20% sucrose and OCT compound (Sakura Finetek) at 4 °C overnight. The specimens were embedded in OCT compound, frozen in liquid nitrogen and sectioned at 12-μm thickness. The sections were mounted on amino silane-coated slide glasses (Matsunami Glass). Washed slides were incubated with 5% FBS, 1% Triton in PBS for 1 h at room temperature, then incubated with primary antibody in 1% FBS, 0.1% Triton-X in PBS overnight at 4 °C. The slides were washed, then incubated with secondary antibody for 1 h at room temperature. The washed slides were mounted and observed as described above. For staining of Scp3 proteins, ESCs were fixed and stained as described [47] . The stained cells were observed under Leica AF6000 system. Immunoprecipitation Antibodies were bound to Protein G Dynabeads (Invitrogen 100.07D) according to the manufacturer’s instruction. Cells were lysed with LS buffer [57] (1 × DPBS, 0.1% NP-40) supplemented with complete protein inhibitor (Roche); lysates were subjected to sonication, and clarified by centrifugation. Supernatants were incubated with antibodies bound to Dynabeads for 10 min at room temperature. The beads were washed, and precipitates were eluted according to the to the manufacturer’s instruction. The eluted proteins were analysed on western blots. Chromatin immunoprecipitation ChIP experiments were carried out as described [58] with some modification. Briefly, 5 μg of antibodies were bound to Dynabeads (Protein G (Invitrogen 100.04D) for anti-Max antibodies, M-280 sheep anti-mouse IgG (Invitrogen 112.01D) for mouse monoclonal antibodies) overnight at 4 °C. ESC suspension was fixed with 1% formaldehyde in ES medium for 10 min. After adding glycine, the cross-linked cells were washed, collected in pellets by centrifugation and quickly frozen by liquid nitrogen. The cells were lysed in SDS lysis buffer, and genomic DNA was sheared by sonication (Branson sonifier 250). After centrifugation, the cleared lysates were incubated with antibody-bound Dynabeads overnight at 4 °C. The beads were washed and the chromatin was eluted and subjected to reverse cross-linking. DNA was purified using the Qiagen PCR purification kit, and analysed by real-time PCR using Power SYBR Green PCR master mix (Applied Biosystems) and primers that spanned transcriptional start sites of the genes of interested. The primer sequences are listed in Supplementary Methods . Accession codes: (a) Microarray data have been deposited in Gene Expression Omnibus under the accession code GSE45181 . How to cite this article: Maeda, I. et al . Max is a repressor of germ-cell-related gene expression in mouse embryonic stem cells. Nat. Commun. 4:1754 doi: 10.1038/ncomms2780 (2013).